An extremely low-density human population exterminated New Zealand moa New Zealand moa (Aves: Dinornithiformes) are the only late Quaternary megafauna whose extinction was clearly caused by humans. New Zealand offers the best opportunity to estimate the number of people involved in a megafaunal extinction event because, uniquely, both the Polynesian settlement of New Zealand and moa extinction are recent enough to be dated with a high degree of precision. In addition, the founding human population can be estimated from genetic evidence. Here we show that the Polynesian population of New Zealand would not have exceeded 2,000 individuals before extinction of moa populations in the habitable areas of the eastern South Island. During a brief (<150 years) period and at population densities that never exceeded ~0.01 km −2 , Polynesians exterminated viable populations of moa by hunting and removal of habitat. High human population densities are not required in models of megafaunal extinction. While it is accepted that Polynesian settlers were responsible for the extinction of moa (Aves: Dinornithiformes) [1] , [2] , [3] , by hunting [4] and habitat destruction [5] , the number of people involved remains unclear, as it does for all late Quaternary extinction events. A population in excess of 5,000 individuals has been suggested [4] but accurate estimates of the human population depend on knowledge of the size of the founding population, potential population growth rates and, especially, the duration of the period of human–moa interaction. Uniquely, the Polynesian settlement of New Zealand [6] and moa extinction [3] are recent enough to be precisely (quasi-decadally) dated, and the founding human population estimated from genetic evidence [7] , so the New Zealand event offers the best opportunity to estimate the number of people present during a megafaunal extinction. Founding human population and human population growth rate can be estimated empirically (founding population [7] ) or can be modelled within close limits (growth rates), but estimates of the period of human–moa interaction have ranged from one [3] to several [4] centuries. Estimates of population size at particular times after settlement are less sensitive to founding population size than to growth rate(s) and, critically, to the duration of the period. For New Zealand, the growth rate (or rates, if they varied with changes in the resource base) applied from the time of settlement, should result in the Maori population of ~100,000 estimated in 1769–1770 (ref. 8 ). To provide a best estimate for the Polynesian population present during the extinction process, the dates of human settlement and of moa extinction, and hence the duration of the interaction, must be known with at least quasi-decadal precision. The chronology of human interaction with moa is not understood as well as the abundant archaeological and palaeontological data might allow. We therefore generated independent estimates of the onset and cessation of human interaction with moa from archaeological contexts, and of moa extinction from natural sites in the South Island ( Fig. 1 ), where the interaction between Polynesians and moa was most intense [2] and where the best archaeological [2] , [4] and palaeontological [9] evidence is available. Much of the South Island, one of the largest (~156,000 km 2 ) temperate islands, is mountainous, so a few moa could have persisted for a few decades in remote areas. Dates for moa from two sites on Stewart Island were included, as at least one of those ages is very late and was from an individual that was probably taken to the island from the South Island by early Polynesians [10] . 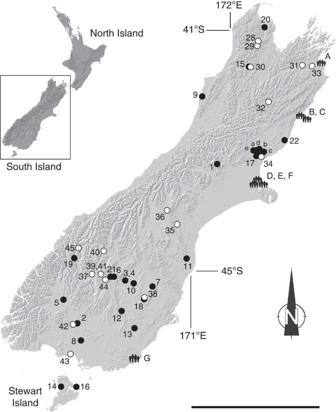Figure 1: Locations of 50 natural deposits and seven archaeological sites on the South Island of New Zealand. Samples were drawn for this study from: a–e, natural sites in North Canterbury; 1–45, additional sites; A–G, archaeological sites. Open symbols, data from ref.50; black symbols, data from this study (a–e, A–G). For sites 1–22, material was identified by bone morphology. Base map courtesy of Department of Geological Sciences, University of Canterbury. Scale bar, 250 km. Figure 1: Locations of 50 natural deposits and seven archaeological sites on the South Island of New Zealand. Samples were drawn for this study from: a–e, natural sites in North Canterbury; 1–45, additional sites; A–G, archaeological sites. Open symbols, data from ref. 50 ; black symbols, data from this study (a–e, A–G). For sites 1–22, material was identified by bone morphology. Base map courtesy of Department of Geological Sciences, University of Canterbury. Scale bar, 250 km. Full size image Determination of the period of Polynesian–moa interactions is complicated by the presence of a large ‘wiggle’ in the terrestrial radiocarbon calibration curve during the 14th century CE. Previous estimates of the time of moa extinction have depended on dating archaeological sites where moa were [4] or had ceased to be [3] a part of the Polynesian diet, and involved relatively few measurements. We therefore adopted a Bayesian approach to dating events, and estimated the time of extinction of moa and of interaction between Polynesians and moa from large, independent, series of calibrated AMS 14 C ages on moa bone collagen from natural (non-archaeological) contexts ( Supplementary Table 1 ), and on moa eggshell from archaeological sites ( Supplementary Table 1 ), respectively. The Bayesian statistical approach [11] , [12] uses the probability distributions of calibrated calendar ages of radiocarbon ages to generate a probability distribution for the cessation of deposition and hence the absence of moa in the local environment. Another approach [13] is to use the number and frequency of dates in a series, weighting the later dates more heavily, to infer when a species actually went extinct, as opposed to assuming, as in the Bayesian analysis, that the youngest available radiocarbon date represents the last appearance of the species. The range of dates yielded by a radiocarbon age is taken into account by incorporating a sigma approximating the age range given by the calibrated date. However, the method requires that the sigma has equal positive and negative ranges, which is very rare for calibrated ages, and it also does not consider the varying date probability within the range given by the calibration curve. Unfortunately, a large ‘wiggle’ in the calibration curve in the 14th century CE results in strongly bimodal probability distributions for the calibrated age ranges and generates 1 σ ranges of 80–100+ years. Both factors make it difficult to estimate the frequency of calendar dates in the decades leading up to the extinction and to determine which should be given higher weighting. We therefore generated large series of radiocarbon ages for both the presence of moa and for the period of interaction between Polynesians and moa and relied on the high number of dates to provide robust probability distributions for moa extinction and for the early human period in New Zealand. There is no archaeological record of Polynesian settlement of New Zealand indisputably older than the Kaharoa eruption of Mount Tarawera (central North Island), which has been assigned a wiggle-match age of 1314±6 years CE [6] . The earliest well-dated occupation, at Wairau Bar in the north-eastern South Island [14] , dates to near the beginning of the 14th century [14] . Evidence of intense human predation on moa there, and at other early archaeological deposits, includes multi-hectare arrays of ‘moa ovens’ [2] , [15] , but most 14 C ages on archaeological sites in New Zealand are on materials with the potential for unknown inbuilt age (for example, charcoal) or subject to marine reservoir effects, which result in large calibrated age ranges [16] . Estimates for the founding Polynesian population in New Zealand, on the basis of analysis of the mtDNA haplotypes of the present Maori population, range from ~70 women [17] to ~170–230 women (~400 individuals) [7] . Despite concerns [18] that the power of such analyses may have been reduced by the effects of a sharp decline in the Maori population after European settlement, the estimate of ~400 individuals accords with oral traditions on the number and carrying capacity of voyaging canoes that reached New Zealand. Just over 450 years later, the population had reached at least 100,000 (refs 8 , 19 ). On the basis of Bayesian analyses of large series of calibrated radiocarbon ages on moa from natural sites and moa eggshell from archaeological sites, constrained by the date for the pre-settlement Kaharoa eruption, we show that Polynesians settled in New Zealand in the early 14th century CE, and that moa went extinct in the early- to mid-15th century CE. At historically reasonable population growth rates, we show that, starting from a genetically estimated founding population of 400 individuals, the Polynesian population of New Zealand during the period of moa exploitation would not have exceeded 2,000, at a density of ~0.01 km −2 . A small population of humans with a basic toolkit of stone tools and fire could, therefore, rapidly eliminate a megafauna by hunting and habitat destruction. Large human populations need not, therefore, necessarily be postulated in the models of megafaunal extinction elsewhere. Period of interaction of Polynesians and moa The Bayesian probability distributions for the start and end of Polynesian interaction with moa (hence the duration of that interaction) are shown as Start and End, respectively, in Fig. 2 . The 68% HPD (highest density of the Bayesian posterior, P =0.681) for the onset of Polynesian exploitation of moa eggs was 1301–1316 CE, and for the cessation 1404–1410 CE (HPD, P =0.657): the 95% HPDs were 1294–1330 CE and 1401–1415, respectively ( Fig. 2 ). The mean span of the sequence of moa egg consumption was 97.02 years ( Fig. 3 ). Comparing the periods of highest probability for the Kaharoa eruption and the onset of moa egg consumption would narrow the probable settlement date for the South Island to somewhere in or after the range 1308 to 1316 CE (yellow bar in Fig. 2c ). 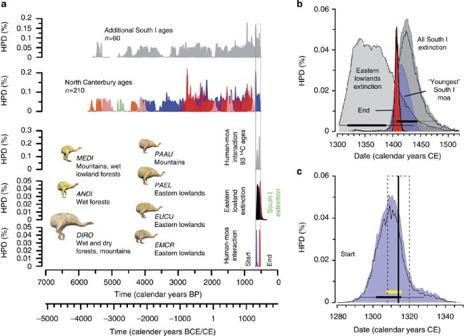Figure 2: Bayesian chronologies for moa extinction and the period of interaction of humans with moa in the South Island of New Zealand. (a) Bayesian highest probability distributions (HPDs) (Datelab V3.512) for 270 natural (bone collagen) and 93 archaeological (eggshell)14C ages on moa; additional South Island, 60 AMS and gas count14C ages (σ≤70 years) from 45 natural sites throughout South Island; North Canterbury, 210 AMS14C ages (σ≤70 years) from five natural sites in North Canterbury (red, Bell Hill Vineyard; blue, Pyramid Valley; pink, Glenmark; orange, Rosslea; green, Glencrieff); human–moa interaction, HPDs for 9314C AMS ages on moa eggshell from seven archaeological sites. Eastern lowland South Island and South Island extinction: black, HPD for moa extinction in the eastern lowlands; red, HPD for moa extinction in South Island. Human–moa interaction: Start, beginning of exploitation period; End, end of exploitation of moa eggs; both based on 9314C ages. Grey outline encompasses period of moa–Polynesian interaction. BCE/CE and BP timescales apply to all distributions. (b) HPDs for moa extinction in eastern lowlands of South Island (distributions as ina); 68% (thick lines) and 95% (thin lines) confidence intervals for whole South Island and eastern lowland extinctions; results of two analyses (shaded and thin line) shown for each; blue, ShCal13 calibration (OxCal 4.2; ref.21) distribution forPachyornis australis(OxA20287), Bulmer Cavern, Mount Owen, ~1,500 m, north-western South Island20. (c) two HPDs (shaded, thin line) for start of Polynesian exploitation of moa eggs in the eastern South Island versus wiggle-match age distribution (dashed box) for Kaharoa event6, centred on 1314 CE (solid line); confidence intervals, start, 68% (thick line), 95% (thin line); thick yellow line, overlap in estimates of start of human–moa interaction moa and date of Kaharoa eruption. MEDI,Megalapteryx didinus; ANDI,Anomalopteryx didiformis; DIRO,Dinornis robustus; PAAU,Pachyornis australis; PAEL,P. elephantopus; EUCU,Euryapteryx curtus; EMCR,Emeus crassus. Figure 2: Bayesian chronologies for moa extinction and the period of interaction of humans with moa in the South Island of New Zealand. ( a ) Bayesian highest probability distributions (HPDs) (Datelab V3.5 12 ) for 270 natural (bone collagen) and 93 archaeological (eggshell) 14 C ages on moa; additional South Island, 60 AMS and gas count 14 C ages ( σ ≤70 years) from 45 natural sites throughout South Island; North Canterbury, 210 AMS 14 C ages ( σ ≤70 years) from five natural sites in North Canterbury (red, Bell Hill Vineyard; blue, Pyramid Valley; pink, Glenmark; orange, Rosslea; green, Glencrieff); human–moa interaction, HPDs for 93 14 C AMS ages on moa eggshell from seven archaeological sites. Eastern lowland South Island and South Island extinction: black, HPD for moa extinction in the eastern lowlands; red, HPD for moa extinction in South Island. Human–moa interaction: Start, beginning of exploitation period; End, end of exploitation of moa eggs; both based on 93 14 C ages. Grey outline encompasses period of moa–Polynesian interaction. BCE/CE and BP timescales apply to all distributions. ( b ) HPDs for moa extinction in eastern lowlands of South Island (distributions as in a ); 68% (thick lines) and 95% (thin lines) confidence intervals for whole South Island and eastern lowland extinctions; results of two analyses (shaded and thin line) shown for each; blue, ShCal13 calibration (OxCal 4.2; ref. 21 ) distribution for Pachyornis australis (OxA20287), Bulmer Cavern, Mount Owen, ~1,500 m, north-western South Island [20] . ( c ) two HPDs (shaded, thin line) for start of Polynesian exploitation of moa eggs in the eastern South Island versus wiggle-match age distribution (dashed box) for Kaharoa event [6] , centred on 1314 CE (solid line); confidence intervals, start, 68% (thick line), 95% (thin line); thick yellow line, overlap in estimates of start of human–moa interaction moa and date of Kaharoa eruption. MEDI, Megalapteryx didinus ; ANDI, Anomalopteryx didiformis ; DIRO, Dinornis robustus ; PAAU, Pachyornis australis ; PAEL, P. elephantopus ; EUCU, Euryapteryx curtus ; EMCR, Emeus crassus . 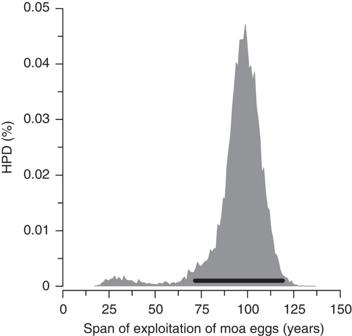Figure 3: The period of exploitation of moa eggs by Polynesians in the eastern South Island of New Zealand. The HPD was based on 93 high-precision AMS14C ages on genetically identified moa eggshell pieces from seven archaeological sites along the eastern coastline of the South Island, New Zealand. Black bar indicates 68% confidence interval. Highest probability is 98.8 years; mean=95.33 years. Full size image Figure 3: The period of exploitation of moa eggs by Polynesians in the eastern South Island of New Zealand. The HPD was based on 93 high-precision AMS 14 C ages on genetically identified moa eggshell pieces from seven archaeological sites along the eastern coastline of the South Island, New Zealand. Black bar indicates 68% confidence interval. Highest probability is 98.8 years; mean=95.33 years. Full size image Moa extinction in eastern lowlands and whole South Island The sample for the eastern lowlands yielded a 68% HPD range for the end of the ‘moa phase’ of 1324 to 1391 CE (HPD, P =0.654), with the 95% HPD lying between 1304 and 1441 CE (HPD, P =0.955; Fig. 2a,b ). Analysis of the 270 ages yielded a 68% HPD for moa extinction in the South Island of 1406 to 1446 CE (HPD, P =0.726), centred on 1426 CE, with a 95% HPD of 1396 to 1480 CE (HPD, P =0.949; Fig. 2 ). The HPD distribution for the end of the moa sequence—extinction in the whole South Island—was robust to repeated analysis. For example, results of a second run are also shown in Fig. 2 , for which the 67% confidence limits (1408 to 1443 CE) and 95.2% limits (1397–1480 CE) differed by 0–3 years from those of the representative run. The Bayesian analyses yield independent models: it is not appropriate to condense them to a joint mean and confidence interval. Similarly, Bayesian analyses generate independent HPDs, and can result in different 1 σ values, as above. The probability distributions do not describe the time course of the event in North Canterbury and the South Island, but are estimates of the probability that extinction occurred in that date range. Youngest dates from natural deposits The ‘youngest’ moa dated from a natural deposit was an individual of Pachyornis australis recovered from Bulmer Cavern ( Fig. 1 ), a cave at ~1,500 m altitude in the remote hinterland of the north-western South Island [20] . An AMS 14 C age on bone collagen from this individual, OxA20287 (564±26 conventional radiocarbon years), was included in the 270 ages used in the Bayesian analysis reported here. Both the Shcal04 and Shcal13 curves in OxCal 4.2 (ref. 21 ) yielded calibrated age ranges of (68.2%) 1404–1428 CE and (95.4%) 1396–1442 CE. The peak probability for its time of death was intermediate between the estimates for moa extinction in the eastern lowlands (on the basis of natural and archaeological sites) and that for moa extinction in the whole South Island ( Fig. 2b ). Youngest dates from archaeological contexts The three youngest eggshell ages included here ( Supplementary Table 1 ) are all early 15th century CE. The eggshell from Monck’s Cave (NZA52715) post-dated moa extinction in the eastern lowlands and may represent a relict population of Euryapteryx curtus in the forests of Banks Peninsula, which survived into the 15th century: forests on the plains and downlands to the west were largely destroyed by fire in the 14th century [5] . The two eggs from Pounawea again could represent a relict population of Dinornis robustus in the remote Catlins Forest of eastern Southland. Several radiocarbon dates on moa remains have been cited [20] as evidence of later survival than is suggested by the rapid extinction model [3] . However, all are either of questionable reliability or lie within the time span modelled in that study. The rapid extinction model [3] suggested that effective extinction took 60–160 years and not 50–100 years as is often cited [20] , [22] . The dates ‘ignored’ [20] in discussion of the rapid extinction model [3] were not actually ‘accepted’ dates but simply were dates that had not been (at that time) shown to be unreliable but which were believed to be so on the basis of the following. Each of the three moa bone dates cited [20] as being ‘accepted’ dates that were not included in the rapid extinction model [3] were processed before 1990. The material used for these ages is difficult to date reliably, and the protocols that would be used now for such materials were not developed until well into the 1990s (ref. 23 ). The Ototara date (NZ754, processed in 1965) has a standard error of ±70 years, at the limit of those included in this paper, and has a likelihood range at 95% consistent with the rapid extinction chronology. The Tumbledown Bay date (NZA338), has a larger standard error (±85 years) and, taken together with the other six dates from the site, is consistent with a date of occupation in the 15th century, the first half of which lies within the chronology of the rapid extinction hypothesis [3] . The Shag River Mouth date (NZ754) is nearly 200 years later than the date of occupation accepted for the site on the basis of a large suite of radiocarbon dates, which otherwise place the date of the site ‘well within the fourteenth century’ [24] . The date was rejected in a later review [23] as being one of a group of dates that the author of the review described as ‘suspect’. The two eggshell dates cited [20] , Wk2604, Shag River Mouth, conventional radiocarbon age (CRA) 570±45 years BP (95.4%, 1319–1451 CE, δ 13 C=11.4,) and Wk2417, CRA 560±45 years BP (95.4%, 1320–1445 CE, δ 13 C=15), are almost identical to the age on the youngest moa included in the Bayesian analyses and their calibrated ages are consistent with the rapid extinction hypothesis. Their inclusion in the analysis would not materially change the results. Polynesian population growth The models suggest that, for all reasonable growth rates of the Polynesian population from its initial size ( Figs 4 and 5 ), the population did not reach 2,000 individuals before 1400 CE ( Fig. 6 ), and was unlikely to be >1,500 during the peak period of moa exploitation. Hence, the population densities for the South Island, for the eastern South Island, and for both main islands during the moa hunting period were among the lowest recorded for any recent hunter–gatherer culture ( Fig. 7 ). 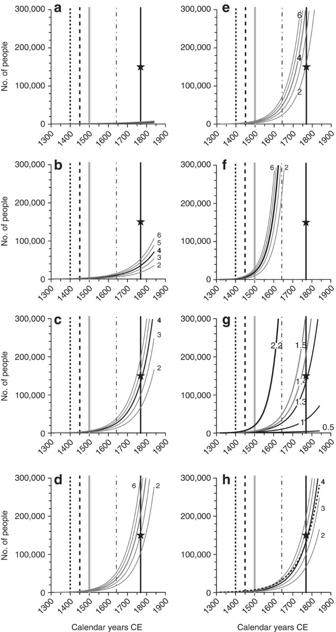Figure 4: Basis of choice of human annual population growth rates used in model for whole prehistory. Population growth at different annual rates during Polynesian prehistory of New Zealand from founding populations of 200, 300,400, 500, 600 individuals (shown as 2, 3,4, 5, 6) at annual rates of: (a) 0.5%; (b) 1.0%; (c) 1.3%; (d) 1.4%; (e) 1.5%; (f) 2.2% continuing after 1400 CE (extinction of lowland populations of moa); (g) population growth for founding population of 400 individuals at the same annual growth rates, as shown; (h) 1.3%, with growth at 2.2% to 1400 CE and 1.1% thereafter indicated by dashed line. Polynesian population in mid 17th century indicated by black star; short dash vertical line, extinction of eastern lowland moa populations; long dash vertical line; extinction of moa in South Island; thick grey vertical line, start of hill fort building; thin chain line, visit by Tasman; black line, first visit by James Cook. Figure 4: Basis of choice of human annual population growth rates used in model for whole prehistory. Population growth at different annual rates during Polynesian prehistory of New Zealand from founding populations of 200, 300, 400 , 500, 600 individuals (shown as 2, 3, 4 , 5, 6) at annual rates of: ( a ) 0.5%; ( b ) 1.0%; ( c ) 1.3%; ( d ) 1.4%; ( e ) 1.5%; ( f ) 2.2% continuing after 1400 CE (extinction of lowland populations of moa); ( g ) population growth for founding population of 400 individuals at the same annual growth rates, as shown; ( h ) 1.3%, with growth at 2.2% to 1400 CE and 1.1% thereafter indicated by dashed line. Polynesian population in mid 17th century indicated by black star; short dash vertical line, extinction of eastern lowland moa populations; long dash vertical line; extinction of moa in South Island; thick grey vertical line, start of hill fort building; thin chain line, visit by Tasman; black line, first visit by James Cook. 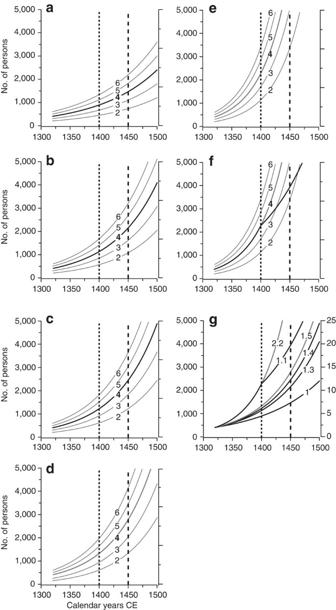Figure 5: Human population growth at different annual rates during period of moa hunting. Models of human population growing from founding populations of 200, 300,400, 500, 600 people (shown as 2, 3,4, 5, 6) at annual rates of: (a) 1%; (b) 1.3%; (c) 1.4%; (d) 1.5%; (e) 2.2%; (f) 2.2% then 1.1% after 1400 CE (extinction of lowland populations of moa); (g) population growth for founding population of 400 individuals, as used in model presented in paper, at annual growth rates as shown. Short dash vertical line, extinction of eastern lowland moa populations; long dash vertical line; extinction of moa in South Island. Full size image Figure 5: Human population growth at different annual rates during period of moa hunting. Models of human population growing from founding populations of 200, 300, 400 , 500, 600 people (shown as 2, 3, 4 , 5, 6) at annual rates of: ( a ) 1%; ( b ) 1.3%; ( c ) 1.4%; ( d ) 1.5%; ( e ) 2.2%; ( f ) 2.2% then 1.1% after 1400 CE (extinction of lowland populations of moa); ( g ) population growth for founding population of 400 individuals, as used in model presented in paper, at annual growth rates as shown. Short dash vertical line, extinction of eastern lowland moa populations; long dash vertical line; extinction of moa in South Island. 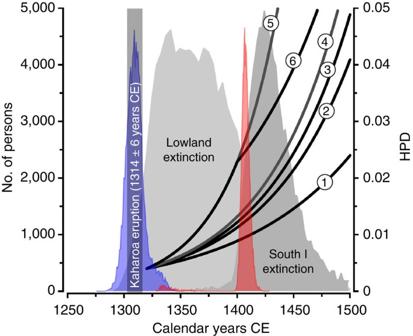Figure 6: The human population in early New Zealand in relation to timing of key events. Human population increases from a founding population of 400 individuals are shown for annual rates of growth (left axis) of:1, 1%;2, 1.3%;3, 1.4%;4, 1.5%;5, 2.2%;6, 1.1% after 1400 CE. Events shown by Bayesian HPDs (right axis) for extinction in eastern lowlands (light grey) and whole South Island (dark grey) based on 21014C ages from five North Canterbury sites, and 27014C ages on moa from 50 natural sites, respectively; HPDs for onset (blue) and cessation (red) of consumption of moa eggs based on 9314C ages on moa eggshell pieces from seven eastern South Island Polynesian occupation sites; age of Kaharoa eruption, 1314±6 years CE6. SeeFigs 4and5for derivation of growth rates. Full size image Figure 6: The human population in early New Zealand in relation to timing of key events. Human population increases from a founding population of 400 individuals are shown for annual rates of growth (left axis) of: 1 , 1%; 2 , 1.3%; 3 , 1.4%; 4 , 1.5%; 5 , 2.2%; 6 , 1.1% after 1400 CE. Events shown by Bayesian HPDs (right axis) for extinction in eastern lowlands (light grey) and whole South Island (dark grey) based on 210 14 C ages from five North Canterbury sites, and 270 14 C ages on moa from 50 natural sites, respectively; HPDs for onset (blue) and cessation (red) of consumption of moa eggs based on 93 14 C ages on moa eggshell pieces from seven eastern South Island Polynesian occupation sites; age of Kaharoa eruption, 1314±6 years CE [6] . See Figs 4 and 5 for derivation of growth rates. 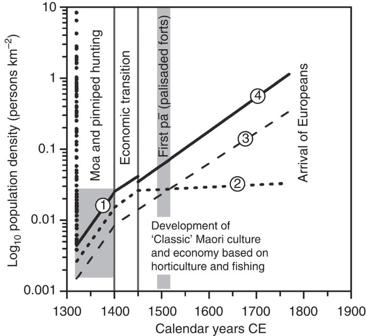Figure 7: Human population densities through New Zealand prehistory. Densities calculated assuming 2.2% annual growth rate from a founding population of 400 individuals until 1400 CE, then annual growth rate of 1.1% after elimination of megafauna. 1, South Island lowlands; 2, all South Island, with movement to North Island after moa extinction; 3, both South and North Islands; 4, North Island after 1400 CE. Black symbols at 1320 CE indicate population densities of hunter–gatherer populations in 20th century31. Shaded rectangle, human population densities during main period of moa hunting, ending at 1400 CE: moa extinction in South Island by 1450 CE. Full size image Figure 7: Human population densities through New Zealand prehistory. Densities calculated assuming 2.2% annual growth rate from a founding population of 400 individuals until 1400 CE, then annual growth rate of 1.1% after elimination of megafauna. 1, South Island lowlands; 2, all South Island, with movement to North Island after moa extinction; 3, both South and North Islands; 4, North Island after 1400 CE. Black symbols at 1320 CE indicate population densities of hunter–gatherer populations in 20th century [31] . Shaded rectangle, human population densities during main period of moa hunting, ending at 1400 CE: moa extinction in South Island by 1450 CE. Full size image Kaharoa eruption date versus 1280 CE for human settlement Most recent commentary on the date of human settlement of New Zealand agrees that no archaeological horizons have been found sealed beneath the Kaharoa Tephra [16] , [25] . Although this has now been dated using high-precision wiggle-match methodology to 1314±6 (1 σ ) CE [6] , there is some reluctance to move on from the 1280 CE date estimated for the earliest well-dated site of Wairau Bar [26] . It has been suggested [27] , [28] that changes to the vegetation in several sediment profiles show that human settlement may have begun before the Kaharoa Tephra, and that the time is consistent with the 1280 CE date proposed for Wairau Bar [26] . However, non-archaeological data have been used in the past [29] , [30] to produce erroneous results [16] , [26] . In the absence of any unequivocal archaeological evidence for pre-Kaharoa settlement, 1314±6 CE should be taken as a TPQ for sustained human settlement in New Zealand. The new quasi-decadal-scale chronology for the Polynesian settlement of New Zealand and the anthropogenic extinction of moa, on the basis of the agreement between the independent chronologies for moa extinction (from the largest suites of 14 C ages ever applied to a megafaunal extinction), and for Polynesian settlement (constrained by the eggshell chronology and the defining Kaharoa eruption) set a limit on the period of human–moa interaction and hence on the size of the human population at the end of the period. The agreement in timing and order of occurrence of these independent estimates of when the events defining the period of moa exploitation took place provide strong support for the new chronology, and also converge on the expectations of the rapid extinction model [3] . The estimated human population size and density during the course of the extinction process could then be compared with those of recent populations of hunter–gatherers [31] . The early Polynesian settlers of the South Island are treated here as hunter–gatherers despite their long history of a horticulture-based culture, because of abundant evidence for significant exploitation of wild land and sea foods and sparse evidence for early gardening in the north-eastern South Island and none south of Banks Peninsula. Population growth during the first century of occupation would, therefore, have been sustained largely by a reversion to hunter–gatherer economics, as when other cultures have encountered climates inimical to maintenance of their farming [32] , especially in the presence of abundant natural food resources. After having stable—or even slightly increasing—populations for the previous several thousand years [1] , moa became extinct in the South Island, as a result of hunting and habitat destruction [2] , [3] , [5] , before 1446 CE, 120 years after the start of the archaeological record in New Zealand [4] . Moa populations were low in the mountainous and wet western areas [9] , [33] , so for humans to have eliminated their populations there in a few decades would not have been as difficult as might be imagined. For example, Polynesians had reached the remote alpine Takahe Valley (45°17′24′′S, 167°39′42′′E) and butchered an upland moa there by middle of the 14th century (NZA2227) [34] . European gold prospectors explored all but the most remote valleys between 1860 and 1880. The extinction across the entire South Island took at the most five moa generations [9] and was substantially complete within four human generations, insufficient time for the birds to develop anti-predation strategies [35] . It was during this period that the drier eastern forests of the South Island were removed by anthropogenic burning and replaced by tussock grasslands [5] , removing the most productive moa habitat, which contained the most diverse and densest moa populations [3] , [9] . For the eastern South Island, where humans were actively hunting moa throughout the 14th century, the independent natural and archaeological chronologies gave the same extinction period. This agreement, the contemporary elimination of most moa habitat in the area [5] and the number of samples from sites preserving bird material through to the present, suggest that there would be no significant Signor–Lipps effect, with moa surviving beyond the probability distributions for local extinction. Similarly, the convergence of radiocarbon ages on purported ‘last’ or ‘youngest’ moa [20] , [36] in the first half of the 15th century, and the absence of moa remains in archaeological sites throughout the South Island younger than that time, both suggest that there were no survivors beyond the probability distribution for whole South Island. Similarly, it is unlikely that, given the similar available dates of last occurrence and the lower numbers of moa living in the lower productivity multi-tier forest that dominated in the North Island [3] , [9] , moa survived later there than in the South Island. The loss of resources and an increasing population drove Polynesians to start building forts to defend horticultural resources within two centuries of settlement ( Fig. 6 ). The large number of 14 C ages allows the definition of a remarkably brief period between human arrival and complete megafaunal extinction in New Zealand, which contrasts sharply with the less clear-cut histories of extinctions in the Northern Hemisphere and Australia [35] , for both of which adequate dating materials are scarce by comparison. The North American event took several thousand years [37] , long enough for the development of new hunting tool kits [38] . Other classic megafauna such as mammoths [39] , [40] and giant deer [40] survived well into the Holocene in peripheral areas, long after humans had recovered their pre-glacial distributions. Polynesians and moa co-existed for, at the very most, 150 of the 450 or so years between settlement and the start of continuous European presence, or roughly one-quarter of the total prehistoric period. In a global context, Polynesians were in sole occupation of New Zealand for ~3% of pre-European Native American history and ~1% of the pre-European Aboriginal history of Australia. The extinction events on those continents were, even if they played out over several centuries or a few millennia, followed by proportionately much longer periods of human presence. Most of the growth in their human populations would have taken place during the period when both the people and the environment were adapting to the loss of the megafauna. Human population sizes during the initial, comparatively ill-defined, stages of human occupation of America and Australia are little known; but in both, the effects were seemingly out of proportion to the size of the human populations. The Polynesian population of New Zealand reached at the most 2,000 individuals by the time of moa extinction ~120 years after settlement, and it was <1,500 during the period of most intense exploitation and habitat removal. Even allowing for moa being long-lived [9] (‘K-selected’) birds with protracted growth [41] and low reproductive rates [9] , [42] and their being naive to human predation [3] , their extinction was caused by a remarkably low number of people. Although the hunting pressure was very high, evidenced by the number of moa in South Island archaeological sites [4] matching estimates for the standing crop of moa [1] , moa extinction was not an instance of ‘overhunting’. The demographics of long-lived vertebrates are such that for even a stable or increasing population [1] , a slight reduction in adult survivorship by the onset of low-level human predation leads inevitably to extinction [3] . In a New Zealand environment that lacked large mammalian predators, the arrival of a new efficient predator [43] sealed their fate [43] . The extinction of moa in New Zealand provides a unique window into what might have happened in the critical decades and centuries that followed the arrival of tiny populations of humans among megafauna elsewhere. Sampling Bone samples from the North Canterbury sites were collected from the mid-shaft of the tibiotarsus and subdivided for the different analyses. Gelatin samples were extracted and purified by IsoTrace New Zealand Ltd, Dunedin, New Zealand (samples AD152, AD153, AD154, AD155, AD156, AD157) and Isolytix Ltd (remainder, same process and operator throughout as Isolytix Ltd took over part of the commercial activity of IsoTrace New Zealand Ltd). Radiocarbon dates on moa bone All but one of the AMS 14 C ages for the North Canterbury samples were measured at the Rafter Radiocarbon Laboratory, GNS Science, Lower Hutt, New Zealand, on gel samples prepared as above. One radiocarbon age was determined by Beta Analytic, Florida. Samples from 209 genetically identified moa of four taxa from North Canterbury are listed in Supplementary Table 1 . Ages from other sources [2] , [10] , [33] , [44] , [45] , [46] , [47] , [48] used in the analyses, including 29 ages for morphologically identified material from the rest of the South Island, 32 ages on genetically identified individuals of Pachyornis elephantopus and P. australis from sites throughout the South Island, and 93 ages on genetically identified moa eggshell pieces from seven archaeological sites are listed in Supplementary Table 1 . All radiocarbon ages were calibrated using the most recent Southern Hemisphere curves, using DateLab 3.5 (ref. 12 ) or OxCal 4.2 (ref. 21 ). Bayesian statistical analyses The Bayesian calibrations followed a phase model using a Metropolis–Hastings MCMC sampler [11] as implemented in DateLab 3.5 (ref. 12 ). All dates were treated as coming from a phase occurring as a single series. Within that phase there were no prior constraints on the relative age of any of the dates. The analysis was made to estimate the date at which the dated events occurred and to provide age estimates for the phase of activity within which the dated events took place (conventional radiocarbon ages are given in Supplementary Table 1 ). The analysis assumes that the date of interest is when moa ceased to be available for deposition in natural sites, that is, the date of the end of the phases of moa presence within the catchment areas of each of the date sets. Each of the date sets ( Supplementary Table 1 ) was run 10 times with sample step sizes varying between 10,000 and 100,000 steps (in 10,000-step increments), collecting 30,000 samples per run, to ensure that there were no sampling artefacts in the results. The results can be regarded as free of sampling artefacts. Representative model parameters for the 210-date set were: Burn 1,000; MaxOffsetForAutocorrelation 100; MaxRange 5,700; Random Seed 1804395497; Sample Interval 10,000; Samples 30,000; TAQ 300; TPQ 6,000; Dates 210; Phases 1. For the 270-date set, model parameters were: Burn 1,000; MaxOffsetForAutocorrelation 100; MaxRange 6,289; Random See d 1.4E+09; Sample Interval 5,000; Samples 10,000; TAQ 333; TPQ 6,622; Dates 270; Phases 1. Period of Polynesian interaction with moa To refine the period of moa–Polynesian interaction, we subjected AMS 14 C ages on 93 genetically distinguished [49] pieces of moa eggshell recovered from seven early Polynesian sites covering the whole eastern seaboard of the South Island to Bayesian statistical analysis ( Supplementary Table 1 ). Moa eggshell is an excellent, short-life dating material [26] that also defines the presence of female moa and therefore, potentially, of a breeding population. All the AMS 14 C ages on moa eggshell from archaeological sites were measured at the Rafter Radiocarbon Laboratory, GNS Science, Lower Hutt, New Zealand [14] . Extinction times for moa For the eastern lowlands, the area of highest human activity, we performed Bayesian statistical analysis on 210 AMS 14 C ages (with 1 σ measurement errors <70 years) from five non-archaeological sites in North Canterbury, an area with substantial evidence for early Polynesian occupation [2] ( Fig. 2a , Supplementary Table 1 ). For the extinction of moa in the whole South Island, we used ages younger than 5,000 years (209 from North Canterbury series), plus 32 (including the geologically youngest moa known so far from natural contexts [20] ) on genetically identified Pachyornis [50] , and a further 29 from the literature [2] , [10] , [33] , [44] , [45] , [46] , [47] , [48] (again with measurement errors <70 years), on individuals identified by their morphology ( Supplementary Table 1 ). The dated specimens were from five sites in North Canterbury, 43 sites distributed throughout the South Island and two on Stewart Island ( Fig. 1 ). Polynesian population growth To determine the human population during and at the end of the period of moa exploitation, we modelled population growth for the period between Polynesian settlement and European landing, assuming both constant rates and higher rates during the initial period. Assuming higher rates during the early Polynesian period takes into account the possibility of higher fecundity and survivorship while substantial resources of protein and fat were available from pinnipeds and large birds. Annual growth rates of Neolithic societies have been estimated at ~0.1% (ref. 51 ) up to 0.4–1.3% (ref. 52 ), up to 1.1% in early modern, pre-industrial, England [53] ; and current population growth rates are 1.5–2.2% (ref. 52 ). Rates of population increase of 0.5, 1.0, 1.3, 1.4, 1.5 and 2.2% were therefore applied, to cover the range of reported values. Founding populations were set at 200, 300, 400, 500, 600 individuals, covering the range of values estimated from genetic evidence [7] . To ensure growth rates that would avoid underestimating the Polynesian population of New Zealand at moa extinction, the population estimated by James Cook in 1769 (ref. 8 ), was increased by 50% to 150,000, indicated by the black star in Fig. 4 , which accords with the mid-range of an earlier estimate (ref. 54 ). In addition, a scenario in which the population growth rate fell from a maximal 2.2 to 1.1% after 1400 CE, on the extinction of lowland populations of moa (and elimination of readily-accessible pinniped populations, which disappear from the archaeological record at about the same time as moa) was included. The population growth rates used could be achieved with mean ages to parturition of 20–25 years and four to six offspring [19] and are consistent with other models of population growth in prehistoric New Zealand, that were developed on the assumption that settlement took place in ~850 CE [19] . How to cite this article : Holdaway, R. N. et al. An extremely low-density human population exterminated New Zealand moa. Nat. Commun. 5:5436 doi: 10.1038/ncomms6436 (2014).